Evolution of the protein stoichiometry in the L12 stalk of bacterial and organellar ribosomes The emergence of ribosomes and translation factors is central for understanding the origin of life. Recruitment of translation factors to bacterial ribosomes is mediated by the L12 stalk composed of protein L10 and several copies of protein L12, the only multi-copy protein of the ribosome. Here we predict stoichiometries of L12 stalk for >1,200 bacteria, mitochondria and chloroplasts by a computational analysis, and validate the predictions by quantitative mass spectrometry. The majority of bacteria have L12 stalks allowing for binding of four or six copies of L12, largely independent of the taxonomic group or living conditions of the bacteria, whereas some cyanobacteria have eight copies. Mitochondrial and chloroplast ribosomes can accommodate six copies of L12. The last universal common ancestor probably had six molecules of L12 molecules bound to L10. Changes of the stalk composition provide a unique possibility to trace the evolution of protein components of the ribosome. Ribosomes—the ancient, ubiquitous protein factories—consist of ribosomal RNA and ribosomal proteins (r-proteins). The sequence and structure of rRNA is extremely well conserved, which allows using the rRNA sequence for construction of phylogenetic trees and analysis of phylogenetic relationships and evolution. Also the sequence and the stoichiometry of r-proteins, which are usually present in one copy per ribosome, are highly conserved. The only r-protein that is present in multiple copies is L12, a protein of the large ribosomal subunit, which is part of the so-called L12 stalk of the ribosome (in bacteria and archaea, or P-stalk in eukaryotes). The L12 stalk entails ribosomal protein L10 (or its archaeal and eukaryotic orthologue P0 in the P-stalk) and multiple copies of protein L12 (P1/P2 in eukaryotes [1] ). The L12 stalk is required for translation, because it recruits to the ribosome the auxiliary translation factors, in particular translational GTPases, such as initiation factor 2, elongation factors Tu and G, and release factor 3 or their eukaryotic homologues [2] , [3] , [4] , [5] , [6] , [7] , [8] , and accelerates GTPase activity of some of them [3] , [9] , [10] , [11] . The mitochondrial homologue of L12, MRPL12, not only has an important role in translation but also regulates the transcription in mitochondria [12] . Variations in the L12 sequence between species provide the specificity for the interactions with translation factors: the replacement of the L12–L10 stalk in Escherichia coli ribosomes with its eukaryotic counterpart (P0/P1/P2 stalk) makes the ribosome to bind eukaryotic, rather than bacterial elongation factor [13] . The evolutionary and functional advantage of having multiple L12 copies is not known; reducing the L12 copy number to just two copies affects both translation efficiency [14] , [15] and accuracy [16] . Ribosomes from E. coli have four molecules of the L12 protein arranged in two dimers bound to one molecule of L10 (refs 17 , 18 , 19 , 20 ). The 4:1 stoichiometry was also found in ribosomes from Bacillus subtilis and Bacillus stearothermophilus [21] . In contrast, ribosomes from Agrobacterium tumefaciens [22] and from a number of thermophilic bacteria, such as Thermotoga maritima , Thermus thermophilus or Thermus aquaticus contain six copies of L12 per L10 (refs 9 , 21 , 23 ), suggesting that the 4:1 stoichiometry of L12:L10 is not universal. This raised the questions of whether stoichiometries other than 4:1 and 6:1 exist in bacteria, whether a given stoichiometry is related to a particular taxonomic group or a specific living environment, or which evolutionary processes resulted in a given stoichiometry. Biochemical and mass spectrometry methods that were used so far to quantify the L12 copy numbers [9] , [17] , [18] , [19] , [20] , [21] , [23] are not suitable for a large-scale screening of hundreds of species. Here we used computational tools to predict the ribosomal L12 stalk composition for a wide range of bacteria, mitochondria and chloroplasts. The predictions for the 8:1 stoichiometry, which has not been seen so far, are validated by mass spectrometry. L12 copy number in bacteria L12 entails two domains, the amino-terminal domain (NTD) and the carboxy-terminal domain, which are connected by a flexible hinge region [24] . The globular carboxy-terminal domain interacts with translation factors [1] , whereas the α-helical NTD is responsible for L12 dimerization and binding to L10. L10 contains eight α-helices and four β-sheets, and the L12 NTD dimers bind to consecutive elements in the C-terminal helix α8 of L10, which comprises α-helical segments separated by bends [9] ( Fig. 1 ). Although in all bacterial species studied so far each segment in helix α8 binds an L12 dimer, the sequence conservation between the segments is too low to allow for a reliable identification of L12 binding in other organisms. However, the copy number of L12 per ribosome depends on the length of helix α8, that is, the number of consecutive helical elements. Thus, secondary structure predictions can be used to locate helix α8 and estimate the number of potential L12-binding segments. This structure-guided approach was first used to predict the 6:1 ratio of L12:L10 in ribosomes from T. maritima [9] and then to analyse bacterial, archaeal and eukaryotic stalks [14] , [25] . Sequence analyses of 28 bacterial, species suggested 4:1 and 6:1 stoichiometries in bacteria [14] , with a tendency towards 6:1 for thermophilic organisms, which may, however, be due to the limited number of sequences studied. 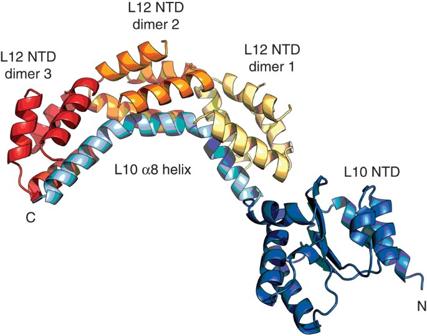Figure 1: Ribosomal protein L10 fromThermotoga maritimain complex with three dimers of the L12 NTD9. L12 carboxy-terminal domains are not shown. Figure 1: Ribosomal protein L10 from Thermotoga maritima in complex with three dimers of the L12 NTD 9 . L12 carboxy-terminal domains are not shown. Full size image To predict L12 copy numbers, >2,000 sequences of r-protein L10 were downloaded from the UniProt database and grouped into 754 characteristic clusters (see Methods ), representing >1,200 different species. For each of these sequences, the length of helix α8 was predicted (see Methods ). The distribution of predicted lengths has a clearly bimodal shape with major peaks corresponding to lengths of helix α8 of 32–33 and 40–42 amino acids ( Fig. 2a ); a few examples for longer α8 helices of around 55 amino acids are also seen. The difference between the two major modes corresponds to exactly one binding segment for an L12 dimer [9] , suggesting that the species with the shorter helix α8 can bind two L12 dimers and those with the longer helix α8 have three L12-binding segments, and thus may have six copies of L12 per L10. The predictions were consistent with the experimentally determined L12 copy numbers for all organisms, where biochemical or mass spectrometry data are available [9] , [21] , [22] ( Supplementary Table S1 ). Phylogenetic analysis suggests that the species with two or three L12-binding segments on L10 are evenly distributed among the tree ( Supplementary Figs S1–S4 ), with 686 sequences with 3 segments and 535 with 2 ( Supplementary Datasets S1, S2 ). 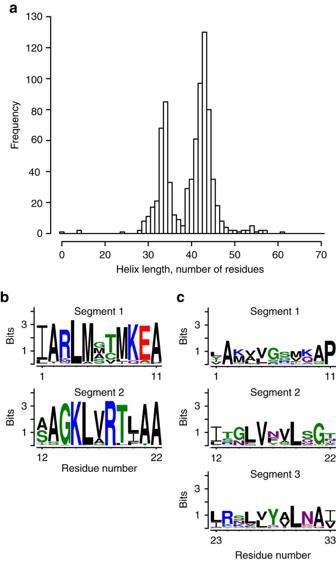Figure 2: L12-binding segments of helix α8 of bacterial L10 proteins. (a) Distribution of the predicted length of helix α8 among L10 proteins. (b,c) Motif logos for the L12-binding segments in helix α8 of L10 sequences, which have more than 50% identity withE. coli(b) and more than 40% identity withT. maritimaL10 (c). Here and later the numbering starts from the fifth amino acid of α8 helix, which corresponds to the start of the first L12-binding segment9. Figure 2: L12-binding segments of helix α8 of bacterial L10 proteins. ( a ) Distribution of the predicted length of helix α8 among L10 proteins. ( b , c ) Motif logos for the L12-binding segments in helix α8 of L10 sequences, which have more than 50% identity with E. coli ( b ) and more than 40% identity with T. maritima L10 ( c ). Here and later the numbering starts from the fifth amino acid of α8 helix, which corresponds to the start of the first L12-binding segment [9] . Full size image Comparison of the sequences of the individual L12-binding segments of L10 provides an insight into the evolution of helix α8 ( Fig. 2b ). For the three L12-binding segments from T. maritima similarity between segments 2 and 3 is significantly higher (motif similarity score 1.18) than between segments 1 and 2 (0.27) or 1 and 3 (0.45). This suggests that the additional, third L12-binding segment has evolved via a duplication of the second segment and subsequent sequence divergence. Sequence clustering analysis ( Supplementary Fig. S5 ) suggests that the first L12-binding segment is more conserved than the other binding segments. Although less conserved than the first segment, the distal segments show a significant degree of sequence similarity to adjacent segments, suggesting that they emerged from consecutive duplication events. Bacteria with eight copies of protein L12 per ribosome Although the length of helix α8 in most bacteria is below 47 amino acids, a few organisms have a particularly long helix α8 comprised of about 55 amino acids with a characteristic pattern of segments that are separated by bends ( Fig. 3 ), suggesting that these ribosomes may bind 8 copies of L12 ( Supplementary Table S2 and Supplementary Fig. S6 ). Most of the organisms that appear to have four potential L12 dimer binding sites are cyanobacteria ( Fig. 4 ), except for two species in the Roseiflexus family. 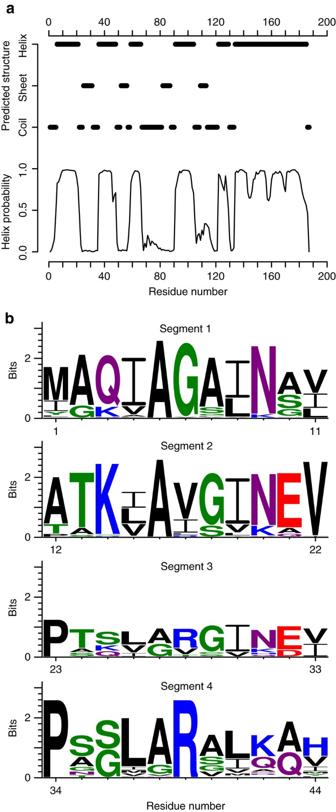Figure 3: Protein L10 fromSynechococcussp. strain JA-3-3Ab (a) Secondary structure predictions of the secondary structure elements (top, α-helices; middle, β-sheets; bottom, random coil) of L10. (b) The confidence of α-helix formation prediction for a given amino acid position in L10; the maximum confidence is set to 1. Amino acid residues are numbered (x axis) starting from the N-terminal fMet. (c) Sequence logos of the L12-binding motifs in helix α8 of L10 fromCyanobacteria. Figure 3: Protein L10 from Synechococcus sp. strain JA-3-3Ab ( a ) Secondary structure predictions of the secondary structure elements (top, α-helices; middle, β-sheets; bottom, random coil) of L10. ( b ) The confidence of α-helix formation prediction for a given amino acid position in L10; the maximum confidence is set to 1. Amino acid residues are numbered (x axis) starting from the N-terminal fMet. ( c ) Sequence logos of the L12-binding motifs in helix α8 of L10 from Cyanobacteria. 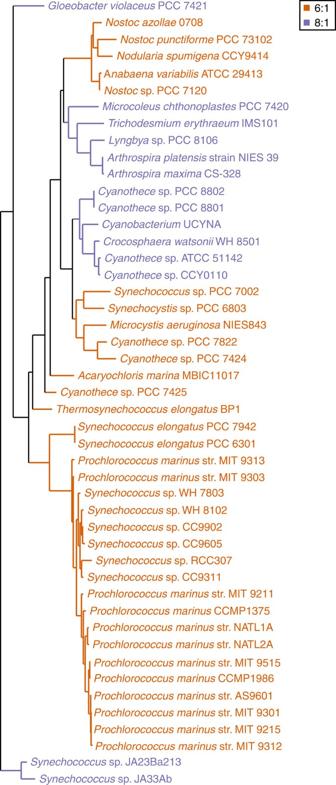Figure 4: Phylogenetic tree of 16S rRNA for cyanobacteria. The predicted L12:L10 stoichiometry is indicated by orange (6:1) or blue (8:1) colour. Full size image Figure 4: Phylogenetic tree of 16S rRNA for cyanobacteria. The predicted L12:L10 stoichiometry is indicated by orange (6:1) or blue (8:1) colour. Full size image To verify the L12:L10 stoichiometry in a species with a particularly long helix α8, we applied a mass spectrometry approach to determine the composition of the L12 stalk of ribosomes purified from Athrospira platensis . We chose A. platensis as a model organism because it can be easily grown in laboratory cultures [26] , and the ribosomes could be prepared using established methods [27] . In contrast to other mass spectrometry approaches that analyse intact macromolecules [21] , the present approach [28] allows the absolute quantification of L12:L10 stoichiometry based on the ratio of peptides obtained by protease digestion, the concentrations of which reflect the concentration of their precursor proteins [29] ( Fig. 5 ), provided protein digestion is complete [30] ( Supplementary Fig. S7 ). To achieve precise quantification, isotopically labelled peptides (absolute quantification peptides, Aqua peptides) were used that had the same sequence and physico-chemical properties as the endogenous peptides to be analysed. Aqua peptides added in known quantities to the digested ribosomal material were used as standards to quantify the mass spectrometric signal intensities in terms of amounts of the respective peptides [28] ( Fig. 5 ). 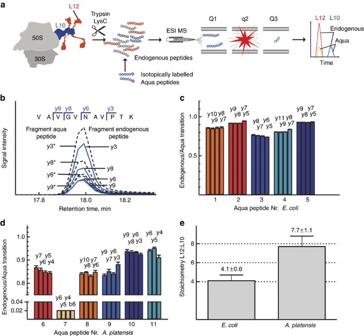Figure 5: Mass spectrometric determination of the L12 copy number in the cyanobacteriumA. platensis. (a) Workflow of a SRM experiment. See text for details. (b) SRM transitions of the respective endogenous and the corresponding Aqua peptide (tryptic L10 peptide 10,A. platensis). Four SRM transitions are depicted. The doubly charged precursor was selected as Q1 mass and the singly charged y9, y8, y6 and y3 fragment ions as Q3 masses. Endogenous peptide (solid lines) and Aqua peptide (dashed lines) co-elute into the mass spectrometer and show identical relative fragment intensities. Peptide ratios were calculated from respective integrated peak areas. (c,d) Endogenous/Aqua peptide ratios analysed by individual transitions. (c) 70S ribosomes fromE. coli(∼65 fmol) were analysed in the presence of Aqua peptides mixed 1:4 (L10:L12), 62.5 fmol L10 peptides. (d) Ribosomes fromA. platensis(∼40 fmol) were analysed in the presence of Aqua peptides (mixed 1:8 (L10:L12), 37.5 fmol L10 peptides). (e) L12:L10 stoichiometry inE. coliandA. platensisribosomes. Figure 5: Mass spectrometric determination of the L12 copy number in the cyanobacterium A. platensis . ( a ) Workflow of a SRM experiment. See text for details. ( b ) SRM transitions of the respective endogenous and the corresponding Aqua peptide (tryptic L10 peptide 10, A. platensis ). Four SRM transitions are depicted. The doubly charged precursor was selected as Q1 mass and the singly charged y9, y8, y6 and y3 fragment ions as Q3 masses. Endogenous peptide (solid lines) and Aqua peptide (dashed lines) co-elute into the mass spectrometer and show identical relative fragment intensities. Peptide ratios were calculated from respective integrated peak areas. ( c , d ) Endogenous/Aqua peptide ratios analysed by individual transitions. ( c ) 70S ribosomes from E. coli ( ∼ 65 fmol) were analysed in the presence of Aqua peptides mixed 1:4 (L10:L12), 62.5 fmol L10 peptides. ( d ) Ribosomes from A. platensis ( ∼ 40 fmol) were analysed in the presence of Aqua peptides (mixed 1:8 (L10:L12), 37.5 fmol L10 peptides). ( e ) L12:L10 stoichiometry in E. coli and A. platensis ribosomes. Full size image Suitable reporter peptides (two peptides for L12 and three for L10) were chosen based on the initial analysis by liquid chromatography tandem mass spectrometry on an Orbitrap mass spectrometer of purified ribosomes that were digested by proteases LysC or trypsin ( Supplementary Table S3 ). For the analysis, peptides were chosen that were unique to L12 or L10, formed quantitatively upon digestion, and did not decay by any side reaction (for example, oxidation or deamidation; Supplementary Table S3 and Supplementary Fig. S7 ). Digested ribosomal material was mixed with synthetic Aqua peptides, and peptides were separated by reversed-phase chromatography and sprayed into a triple quadrupole mass spectrometer. The intensities of both Aqua and endogenous L10 or L12 peptides were monitored by selected reaction monitoring (SRM [30] ; Fig. 5a and see Methods ). In SRM experiments, quadrupole 1 (Q1) selects the defined precursor peptide mass (endogenous or Aqua peptide), q2 is used for gas-phase fragmentation of the selected peptide, and Q3 serves for selecting distinct fragments of the precursor peptide, the so-called ‘SRM transitions,’ which are subsequently detected and quantified. From the amounts of L12 and L10 peptides, the stoichiometry L12:L10 was calculated. As a control, E. coli ribosomes were used for which the L12 copy number is known [1] , [9] , [21] . To obtain reliable results, three to four SRM transitions were chosen for the quantification of each peptide ( Fig. 5b–d and Supplementary Table S3 ). The linearity of the sample signal response in the SRM experiments was established by titrations of each Aqua peptide over four orders of magnitude at constant concentration of endogenous peptides ( Supplementary Fig. S8a,b ). We varied the concentration of either Aqua or sample peptides ( Supplementary Fig. S8c,d ) within a concentration range around a fixed concentration of sample or Aqua peptides, respectively. Knowing the concentrations of the two peptides of L12 and the three peptides of L10 in the digestion mix, we calculated the L12:L10 stoichiometry from six possible combinations of peptides for each titration point. As we found no systematic bias for any of the combinations, we averaged over all titration points and all technical and biological replicates. This approach yielded a L12:L10 ratio of 4.1±0.6 for E. coli (based on 702 independent values; Fig. 5e and Supplementary Dataset S3 ), in agreement with the published values. For purified ribosomes from A. platensis the L12:L10 ratio was 7.7±1.1, suggesting close to four L12 dimers attached to L10, in accordance with the particularly long α8 helix of that organism, as predicted by the computational approach. Notably, not all cyanobacteria included in the computational analysis have a long helix α8, and those with the long helix α8 do not form a monophyletic group ( Fig. 4 ). Given the high sequence similarity in helix α8 for cyanobacteria that have four L12-binding segments ( Supplementary Fig. S6 ), an independent acquisition of the additional segment seems highly unlikely. This suggests that the duplication of the L12-binding segment in helix α8 occurred in a common ancestor of the cyanobacteria. Furthermore, Bayesian ancestral state inference [31] (see Methods ) suggests that the common ancestor of cyanobacteria had a long helix α8, which could accommodate four L12 dimers (calculated probability 0.86). Notably, this kind of analysis does not take into account the sequence similarity among L12-binding motifs, providing an independent indication for a high L12 copy number on the ribosomes of the ancestral cyanobacteria. The shorter L10 variants in some cyanobacteria then would be the result of a later loss of one L12-binding segment. Of the four predicted L12-binding segments of L10 from cyanobacteria, segment 1 is similar (1.36) to segment 1 of helix α8 of L10 from T. maritima sequence family ( Figs 2c and 3b ), which further confirms high conservation between the first binding segments across species. Segments 3 and 4 from cyanobacteria have very similar sequences (1.8), but have significantly lower similarity scores to segments 1 and 2 (0.18–0.72). L12 copy number in mitochondria and chloroplasts With the same computational approach as described above, we analysed the length of helix α8 in the mitochondrial homologue of L10, MRPL10, and in L10 from chloroplasts using all sequences that could be unambiguously assigned as organellar L10 in eukaryotic genomes. In general, mitochondrial ribosomes are quite different from bacterial ones, as they contain many more proteins and less rRNA [32] . The fact that the closest MRPL10 orthologue is L10 from alphaproteobacteria reflects the alphaproteobacterial origin of mitochondria [33] . We analysed MRPL10 sequences from 82 eukaryotes ( Supplementary Table S4 ). The prediction of three L12-binding segments of MRPL10 indicated that mitochondrial ribosomes bind six molecules (three dimers) of L12 ( Fig. 6 ). Similar to mitochondrial ribosomes, chloroplast ribosomes are highly specialized and emerged through an early endosymbiotic event, where a photosynthetic prokaryotic ancestor related to cyanobacteria entered a eukaryotic cell. We analysed chloroplast L10 sequences from 29 species ( Supplementary Table S5 ). All these chloroplast L10 sequences have three L12-binding segments. 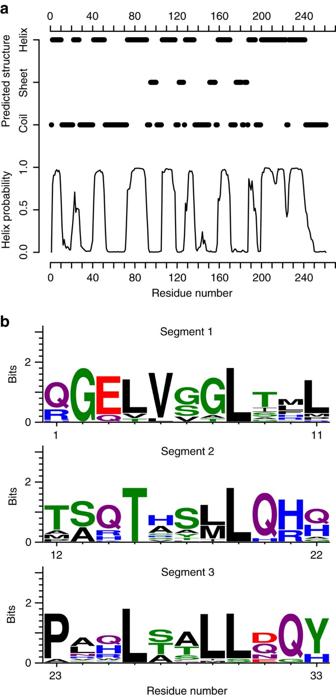Figure 6: L10 from human mitochondrial protein MRPL10. (a) Secondary structure prediction. (b) The confidence of α-helix formation prediction. (c) Sequence logos of the L12-binding segments in helix α8. Figure 6: L10 from human mitochondrial protein MRPL10. ( a ) Secondary structure prediction. ( b ) The confidence of α-helix formation prediction. ( c ) Sequence logos of the L12-binding segments in helix α8. Full size image Emergence of the L12-binding segments The phylogenetic analysis suggests two possible evolutionary scenarios for the change of the L12 copy number, that is, the acquisition or the loss of helix α8 fragments of L10 ( Fig. 7a ). The two possibilities can be distinguished by analysing the phylogenetic tree of L10. In cases where many species predicted to have three L12-binding segments cluster closely together, whereas only a few species in the group have shorter helices α8, we classified the event as a segment loss. Vice versa, if a few members of a phylogenetically related group have a longer helix α8 indicative of binding of six copies of L12, whereas the majority has a shorter helix α8, the event can be classified as acquisition of a segment. Phylogenetic analysis indicated a loss of 11 amino acids in helix α8 of L10 in Deinococcus ( Fig. 7a ), Opitutaceae , Veillonella , Dichelobacter and Methylotenera . In contrast, an acquisition of 11 amino acids seemed to have occurred in Clostridiales ( Fig. 7b ) and in Nitratiruptor . In general, it appears that the loss of a L12-binding segment is the more frequent event. Bayesian approach to ancestral state inference suggested a higher probability (0.67) for helix α8 in L10 of the last bacterial common ancestor to accommodate six copies of L12, rather than four copies (probability 0.33; organisms with eight copies of L12 bound to L10 are too rare to be included in the analysis). 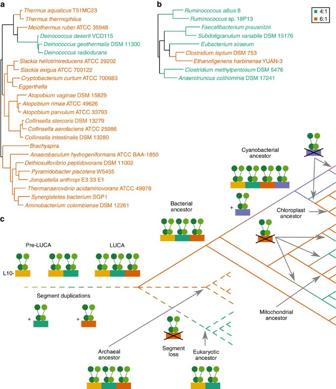Figure 7: Evolutionary scenarios for the emergence of the L12 copy number. (a) Loss of an L12-binding segments in helix α8 of L10. (b) Acquisition of an additional potential L12-binding segment. The phylogenetic trees are based on 16S rRNA sequences. The predicted L12:L10 stoichiometry is indicated by orange (6:1) or green (4:1) colour. (c) A schematic of a proposed evolutionary path. Dashed lines indicate those changes in the L12:L10 copy number for which only limited experimental evidence exists. Figure 7: Evolutionary scenarios for the emergence of the L12 copy number. ( a ) Loss of an L12-binding segments in helix α8 of L10. ( b ) Acquisition of an additional potential L12-binding segment. The phylogenetic trees are based on 16S rRNA sequences. The predicted L12:L10 stoichiometry is indicated by orange (6:1) or green (4:1) colour. ( c ) A schematic of a proposed evolutionary path. Dashed lines indicate those changes in the L12:L10 copy number for which only limited experimental evidence exists. Full size image The origin and evolution of ribosomes are central questions for understanding the emergence of life. It is generally assumed that the ribosome emerged from the RNA world, when the proteins did not exist yet, and RNA acted as catalyst in chemical reactions (for recent reviews see [34] , [35] ). In fact, the peptidyl transferase centre of the ribosome, which appears to be a relic from that ancient time [36] , [37] , is built of RNA [38] , and its activity is not appreciably affected by the r-proteins (for review, see [39] ). The time of adding r-proteins is controversial [36] , [40] . It seems reasonable to assume that the emergence of the L12 stalk proteins is coupled to the evolution of the translation factors and leads to higher speed and fidelity of translation [40] , which is consistent with the important role of L12 in the recruitment of translation factors to the modern ribosome [9] . Very early in evolution, probably only one copy of L12 was present on the ancestral ribosome ( Fig. 7c ). The earliest event that altered the L12 copy number must have been the emergence of the L12 NTD dimerization surface and its binding surface on L10; however, the traces of these stages of ribosome evolution eroded away. It is likely that this first sole binding segment was duplicated early in evolution. In fact, none of the organisms for which genomic data is available so far has L10 with helix α8 so short as to account for only one L12 dimer binding. Rather, the length of helix α8 in most organisms is consistent with binding of two or three L12 dimers, largely independent of the taxonomic group or the living conditions of bacteria. The only exceptions from this ‘four or six copies’ rule are found in cyanobacteria, which show a very long helix α8, indicating binding sites for eight copies of L12. Organisms with a higher potential copy number were not identified. The ribosomes from mitochondria and chloroplasts have three L12-binding segments on L10, suggesting the presence of six L12 copies on those ribosomes. Notably, in all cases where the L12:L10 stoichiometry was determined experimentally, the L12 copy number per ribosome is in excellent agreement with the computationally predicted value ( Supplementary Table S1 ), providing a strong support for the validity of the present computational analysis. Bayesian inference of the ancestral state using the distribution of species with different L12 copy numbers and the sequence analysis of the individual L12-binding segments of L10 from cyanobacteria suggest that in the last bacterial common ancestor the L12 copy number was at least six, whereas the last common ancestor of cyanobacteria had eight copies of L12 per ribosome. As also archaeal ribosomes can bind six copies of L12 (refs 14 , 21 ), it is likely that the hypothetical last universal common ancestor had six copies of L12 ( Fig. 7c ). In this scenario, modern bacterial species with four L12 copies emerged through a loss of one of the three L12-binding segments of helix a8 of L10, whereas, chloroplasts and those cyanobacteria that have six copies of L12 lost one of four segments. One interesting observation is that the sequence of the first L12-binding segment is more evolutionary conserved than the sequences of the other segments. One can hypothesize that the primary structure of the first segment is particularly important for L12 recruitment or the function of the ribosome stalk, thereby limiting the sequence variations, whereas deviations in sequences of other binding segments apparently can be tolerated better. Incidentally, the binding of the L12 dimer to the first segment of helix α8 is stabilized by interactions with the L10 NTD, which are not seen for the more distal dimers [9] . This additional structural constrain may explain the higher degree of sequence conservation in the proximal segment of L10. The distal domains appeared as a result of sequential duplications followed by divergence in the primary sequence of the segments, while retaining their ability to bind L12. The high sequence similarity between the last two binding segments of L10 from cyanobacteria suggests that the additional binding segment resulted from a recent duplication event. The reasons for acquiring multiple copies of L12 and for variable copy numbers of L12 are not known. The high copy number does not correlate with thermophilicity, in contrast to suggestions based on analysis of a limited number of bacterial species [14] , [21] . Multiple copies of the protein may increase the encounter frequency with translation factors, thereby facilitating their recruitment to the ribosome. Kinetic evidence suggests that a complete removal of L12 from E. coli ribosomes decreases the rate of elongation factor Tu binding to the ribosome more than tenfold [9] . On the other hand, ribosomes that have only one L12 dimer are active in translation in vitro [41] . An E. coli strain with mutant L10 that can only bind a single L12 dimer is viable, but shows growth defects and is less efficient than the wild-type strain in initiation and elongation [15] . Ribosomes with four L12 copies (from E. coli ) perform all translation functions with the same speed and efficiency as those with six copies (from M. smegmatis ), both with homologous and heterologous factors [42] . It appears that adaptive selection tends to maintain the stoichiometry in the L12 stalk between four and eight copies of L12. Variations in this range are tolerated without appreciably affecting the activity of the ribosomes, whereas reducing or increasing the copy number beyond these limits would probably lead to reduced fitness of bacteria. Our quantitative analysis of purified ribosomes by mass spectrometry suggests that essentially all potential binding segments on L10 are occupied by L12, which is consistent with the earlier immunoblot analysis of other bacterial ribosomes, for example, from E. coli , T. maritima [9] and M. smegmatis (unpublished data), and mass spectroscopy data [14] , [21] . This suggests that the maximum possible L12:L10 occupancy is sustained in the bacterial cell. In contrast, a mixture of 4:1 and 6:1 stoichiometries was found in the mesophilic archaeon Methanococcus vannielii , suggesting that, in that organism not all binding segments on L10 are occupied by L12. The differences in the stringency of how the stalk composition is maintained may arise from the stability of the stalk and from the regulation of the expression of L10 and L12. The E. coli L10:L12 stalk of the ribosome is very stable, allowing for the dissociation of less than 10% of L12 per hour [9] , [43] . Archaeal stalk may be less stable than in bacteria, resulting in the dissociation of proteins during ribosome purification. The expression of the L10 operon, which codes for both L10 and L12, is controlled by an autoregulation mechanism where the L10:L12 complex inhibits the translation of its own mRNA by binding to the leader preceding the coding sequence [44] ; in addition, although the L10 in the stalk is rather stable, excess free L10 is probably rapidly degraded [45] , thereby maintaining matching relative concentrations of the two proteins in the cell. In archaea, the control mechanisms appear to be different, because the genes encoding L10 and L12 are part of the L1 operon, and the L10:L12 complex does not regulate the expression of the operon [46] . In summary, the present combination of computational predictions and quantitative mass spectrometry provides an insight into the emergence of protein stoichiometry in the functionally important ribosomal L12 stalk and suggests a wide range of stalk compositions—with four, six or eight copies of L12 per L10—on ribosomes from bacteria, mitochondria and chloroplasts. Sequence selection The UniProt database [47] was used as a source for amino acid sequences. L10 and L12 sequences were retrieved using family requests ‘ribosomal protein L10P family’ and ‘ribosomal protein L12P family’, respectively. Sequences with 90% sequence identities were clustered, and each cluster was represented by a single sequence in further analysis. Manual curation included the analysis of sequence completeness and similarity to other sequences. 754 L10 sequences formed the target sample that represented >2,000 individual sequences. Sequence logos were created using WebLogo server [48] , using the chemistry colour scheme. A search of the NCBI database for organellar L10 sequences yielded 82 mitochondrial and 29 chloroplastic sequences that could be unambiguously annotated. The sequences of putative L10 of several plants [49] were not included because of their unclear origin. Helix prediction algorithm As the divergence in sequences precludes the unbiased identification of the potential L12-binding segments based on the sequence comparison, the L12-binding segments were located based on the length of helix α8. The PSIPRED [50] software was used to predict secondary structures. A continuous region with a confidence value for being in a helical conformation of >0.1 and a boundary position confidence of >0.9 was considered to form a helix. The weight of a helical region was calculated as the sum of the confidence values for all of its positions. As helix α8 is the longest α-helix in L10, the helical region with the maximum weight was considered as helix α8. The number of potential L12-binding segments was predicted based on the length of helix α8, with 28–37 amino acids in helix α8 corresponding to two binding segments for the L12 dimer and 39–51 amino acids corresponding to three L12-binding segments. Intermediate cases were re-analysed manually, based on alignments with similar sequences. Motif comparison Motif similarity scores were calculated based on the BLOSUM62 distance score normalized by sequence length. The distance score was calculated for each possible pair of sequences forming different motifs. A median of the corresponding distance score distribution was used as motif similarity score. Sequence clustering of all bacterial helix α8-binding segments was performed using CLANS [51] . Binding segments were located using jackhmmer algorithm [52] . To improve the sensitivity of search, only the C-terminal region of L10 was used starting from ten amino acids upstream of the predicted start of helix α8. Individual segment sequences were extracted from the HMM profile-based alignment. Cyanobacterial binding segments were located manually based on multiple sequence alignment. Supplementary Fig. S5 , illustrating the sequence clustering, was produced using igraph library [53] . Phylogenetic analysis Amino acid sequences for the L10 and L12 families were aligned using T-coffee [54] . Regions corresponding to helix α8 were excluded from the alignments. The phylogenetic trees for L10 and L12 were built using maximum likelihood algorithm implemented in PhyML [55] . The All-Species Living Tree [56] was used as a source for the 16S rRNA tree. Ancestral state inference Ancestral state inference was performed using MrBayes software [31] , [57] , [58] . For the cyanobacterial ancestral state inference, 16S rRNA sequences were collected manually from the NCBI Entrez database. A set of positions was eliminated using Gblocks [59] . T. thermophilus was used as an outgroup species. For the bacterial ancestral state inference (excluding cyanobacteria), 16S rRNA sequences from the All-Species Living Tree [56] project were used. Sequence alignment and position elimination was performed as described above. Archaeal 16S was used as an outgroup. Ribosome preparation A. platensis (strain B-256) cells were grown in Zarrouk’s medium at 35 °C under continuous illumination at 50 μmol photons per m 2 s with 1% (v/v) CO 2 aeration [26] at the Institute of Plant Physiology (Russia, Moscow). Ribosomes from A. platensis and E. coli were prepared as described [27] . Proteolysis of ribosomes All reactions were performed in low-retention reaction cups (Eppendorf). Ribosomes (100 pmol, ∼ 150 μg) in 100 μl buffer A (50 mM Tris–HCl pH 7.5, 70 mM NH 4 Cl, 30 mM KCl, 7 mM MgCl 2 ) were digested by RNase A (5 μg, 0.5 μl; Fermentas) for 3 h at 25 °C. The reaction mixture was lyophilized in a vacuum centrifuge (Speedvac). The pellet was dissolved in 30 μl 1% RapiGest (in 25 mM NH 4 CO 3 ; Waters) and incubated at room temperature for 15 min. For the reduction of cysteines 30 μl 50 mM dithiothreitol (in 25 mM NH 4 CO 3 ; AppliChem) were added and the sample was incubated for 30 min at 60 °C. Alkylation of cysteines was subsequently performed by the addition of 10 μl 100 mM iodoacetamide (in 25 mM NH 4 CO 3 ; Sigma-Aldrich) and incubation for 30 min at room temperature. LysC (0.3 μg in 210 μl 25 mM NH 4 CO 3 ; Roche Diagnostics) was added, followed by an incubation for 3 h at 25 °C. Trypsin (Promega) was added (2 μg in 3 μl) and the sample was digested for 16 h at 25 °C. Formic acid (3 μl 100% formic acid) was added to decompose the Rapigest and incubated for 30 min at 37 °C. Alternatively, the ribosomes were digested with RNase A in the presence of 50% acetonitrile or 2 M urea as described above, lyophilized and then proteolysed as described [30] . Mass spectrometry We have used the selected reaction monitoring (SRM) technique, because it is extensively validated [28] , [60] , sensitive and, unlike the native mass spectrometry, robust and applicable for inhomogeneous samples. This is particularly advantageous for complexes for which no established purification protocol exists and where the stability of the target complex is unknown (for example, ribosomes from an organism which has not been studied in detail). In addition, peptide-based approaches are less restricted than the native mass spectroscopy with respect to detergents, salts and crowding agents used for the complex purification and do not require a sophisticated specialized equipment and software. For each organism, two tryptic peptides of L12 and three peptides of L10 were quantified ( Supplementary Table S3 ). Samples for mass spectrometry analysis were mixed in glass vials in 10% acetonitrile/0.1% formic acid in a final volume of 100 μl. Heavy isotope-labelled Aqua peptides (5 μM) were purchased from Thermo Scientific (guaranteed concentration error of less than 5%) and dissolved in 5% acetonitrile. The effective concentration of Aqua peptides was validated by lyophilizing an aliquot and re-dissolving in 60% acetonitrile/0.1% formic acid. Aqua peptides were premixed in 10% acetonitrile/0.1% formic acid at a concentration of 0.125 μM (L10 peptide) either at a ratio 1:1 ( Supplementary Fig. S8a,b ) or 1:4 (L10:L12, E. coli ) and 1:8 (L10:L12, A. platensis ; Fig. 5e , Supplementary Fig. S8c,d and Supplementary Dataset S3 ). Premixed Aqua peptides and sample were added as indicated. Five microlitre of the sample (containing the absolute amounts of sample or Aqua peptides as indicated) were used for further analysis. Absolute quantification by SRM SRM measurements were performed on a TSQ Vantage Triple Quadrupole mass spectrometer (Thermo Fisher Scientific). Chromatographic separations of peptides were performed on an Easy nLC II Nano LC system (Thermo Fisher Scientific). The peptides were loaded on a self-packed trap column (2 cm length, 150 μm inner diameter, packed with Reprosil-Pur 120 C18 5 μm material (Dr Maisch) with a maximal flow of 10 μl min −1 (buffer B: 2% acetonitrile/0.1% formic acid) limited by a pressure maximum of 200 bar. The trap column was washed with 50 μl under the same conditions. The peptides were eluted by a gradient (35 min) from 2% acetonitrile/0.1% formic acid to 60% acetonitrile/0.1% formic acid from an in-house packed trap column (14 cm length, 75 μm inner diameter, packed with Reprosil-Pur 120 C18 3 μm material (Dr Maisch). The nanoLC was operated at a flow of 300 nl min −1 . Q1 and Q3 were both set to unit resolution (0.7 full width at half maximum). A spray voltage of +1,650 V was used with a heated ion transfer setting of 270 °C for desolvation. The declustering voltage was kept constant at 10 V and the Chromfilter of 10 was used. For each SRM transition, the collision energy was optimized by regular injection of Aqua peptides varying the collision energy (±5) around the theoretical value predicted by the skyline software. SRM transitions for the native peptides were obtained by Q1/Q3 mass transcription, using the expected mass differential from the standard peptides by the Skyline software ( Supplementary Table S3 ). Scheduled transitions were recorded in a time window of 4 min. The cycle time was 3 s and the average dwell time 200–300 ms per transition. The peptide ratios were obtained by peak integration of the individual transitions using the Skyline software ( http://proteome.gs.washington.edu/software/skyline ). The individual transitions show an s.d. of less than 5% and were therefore averaged to yield one peptide ratio. The fact that the individual transitions show identical ratios between endogenous and Aqua peptide, as well as same chromatographic retention time, together with the observation that the different peptides show similar ratios, clearly demonstrates that the detected SRM signal indeed derives from the targeted peptides. In each experiment, 78 individual complex stoichiometries were calculated (48 from the Aqua titration and 30 from the sample titration). For the determination of the complex stoichiometry, three independent biological samples were analysed, each of them in triplicate. Thus, the determined complex stoichiometry for each organism is the average of 702 individual values for the complex stoichiometries that were generated based on 117 individual HPLC runs. How to cite this article: Davydov, I. I. et al. Evolution of the protein stoichiometry in the L12 stalk of bacterial and organellar ribosomes. Nat. Commun. 4:1387 doi: 10.1038/ncomms2373 (2013).